Activity-driven relaxation of the cortical actomyosin II network synchronizes Munc18-1-dependent neurosecretory vesicle docking In neurosecretory cells, secretory vesicles (SVs) undergo Ca 2+ -dependent fusion with the plasma membrane to release neurotransmitters. How SVs cross the dense mesh of the cortical actin network to reach the plasma membrane remains unclear. Here we reveal that, in bovine chromaffin cells, SVs embedded in the cortical actin network undergo a highly synchronized transition towards the plasma membrane and Munc18-1-dependent docking in response to secretagogues. This movement coincides with a translocation of the cortical actin network in the same direction. Both effects are abolished by the knockdown or the pharmacological inhibition of myosin II, suggesting changes in actomyosin-generated forces across the cell cortex. Indeed, we report a reduction in cortical actin network tension elicited on secretagogue stimulation that is sensitive to myosin II inhibition. We reveal that the cortical actin network acts as a ‘casting net’ that undergoes activity-dependent relaxation, thereby driving tethered SVs towards the plasma membrane where they undergo Munc18-1-dependent docking. In neurosecretory cells, Ca 2+ -dependent secretory vesicle (SV) fusion requires docking to the cellular plasma membrane [1] , [2] , [3] . Before docking, most SVs need to undergo translocation from the cytosol to the plasma membrane. The mechanisms governing this transition towards their docking sites determine both the number of release-ready vesicles and the sustainability of the secretion process. During stimulation, the initial round of release is achieved by the fusion of a small number of already docked or primed vesicles [3] , [4] , [5] , [6] , but prolonged stimulation requires the translocation of SVs that are not in the immediate vicinity of the plasma membrane. The cortical actin network plays a major role in regulated exocytosis [2] , [7] and has been shown to interact with SVs in various ways, in particular through the action of myosin molecular motors [8] , [9] . SVs can be tethered to the cortical actin network by myosin VI in an activity-dependent manner [10] , and can also be transported along actin fibres by myosin Va [11] . Recent work has also highlighted a role for myosin II in exocytosis [12] , [13] , [14] , [15] , [16] , [17] , as well as demonstrating its ability to maintain the cortical actin network under tension [18] , [19] , [20] . How these molecular motors act to direct SVs towards their docking sites remains unclear. Here we reveal that secretagogue stimulation promotes a reduction in cortical actin network tension, facilitating the movement of SVs towards the plasma membrane where they undergo Munc18-1-dependent docking. SVs and cortical actin approach the plasmalemma on stimulation To image SV- and F-actin dynamics before and during secretagogue stimulation, bovine chromaffin cells were transfected with the SV marker neuropeptide-Y (NPY)-mCherry and the F-actin marker lifeact-green fluorescent protein (GFP). Time-lapse-total internal reflection fluorescence (TIRF) microscopy was used to image NPY-mCherry-positive SVs and lifeact-GFP-positive actin in the transfected cells. Stimulation using either Ba 2+ (2 mM) [21] , [22] or nicotine (100 μM) led to a coincident albeit transient increase in fluorescence intensity for both lifeact-GFP and NPY-mCherry ( Fig. 1a,b , Supplementary Fig. 1a,b , Supplementary Movie 1 ), which was not observable using widefield illumination ( Supplementary Fig. 1c ). The average change in fluorescence intensity measured 30 s after stimulation with Ba 2+ was 35±2.5% (s.e.m. ; n =10) for lifeact-GFP and 41±2% ( n =10) for NPY-mCherry ( Fig. 1c ). With nicotine stimulation, the average fluorescence intensity increase was 23±2% for lifeact-GFP and 42±15% for NPY-mCherry ( n =5; Supplementary Fig. 1b ). Vehicle treatment did not affect the TIRF fluorescence intensity ( Fig. 1c ). Considering the exponential decay of the evanescent wave penetrating the sample in TIRF illumination, we concluded that both the cortical actin network and SVs translocate closer towards the illumination plane and thus to the basal plasma membrane of the cells. To exclude the possibility of an artifactual increase in fluorescence intensity associated with an overall movement of the cell towards the coverslip, we expressed the plasma membrane marker GFP–glycosyl phosphatidyl inositol (GPI) and found no significant change in fluorescence in the GFP–GPI channel ( Supplementary Fig. 1d ), confirming that secretagogue stimulation promotes translocation of F-actin and vesicles without causing any significant displacement of the GFP–GPI-labelled plasma membrane. 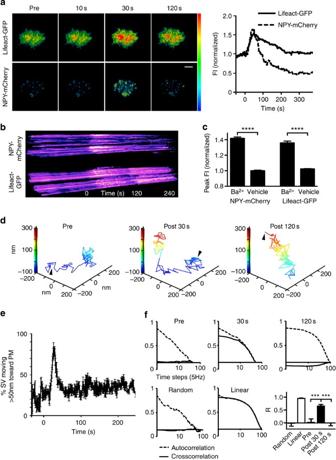Figure 1: SVs undergo highly correlated movement that coincides with cortical F-actin translocation towards the plasma membrane following secretagogue stimulation. (a) Bovine chromaffin cells expressing NPY-mCherry and lifeact-GFP were examined by TIRF microscopy, imaged at 2 Hz and stimulated with Ba2+(2 mM). Fluorescence intensity is depicted in pseudocolour (range: 11,000–28,000 for lifeact-GFP, 2,000–12,000 for NPY-mCherry). Plotted time course of change in NPY-mCherry and lifeact-GFP fluorescence intensity (FI). Scale bar, 5 μm. (b) 3D rendering of vesicle trajectories and actin structures over time, highlighting the simultaneous increase in fluorescence intensity for NPY-mCherry and lifeact-GFP. (c) Average maximum change in fluorescence intensity (normalized to fluorescence intensity before treatment) for Ba2+- or vehicle-treated cells (mean±s.e.m.;n=10). ****P<0.0001 (Student’st-test). (d) 3D SV trajectories before and at indicated time points during stimulation. Colour code indicateszposition. (e) Time course of percentage vesicles moving simultaneously towards the plasma membrane. Scoring was based on the percentage of vesicles that moved more than 50 nm in a sliding 10-s interval. (f) Multi-cross-correlation analysis of lateral vesicle movement before and at indicated time points during stimulation. Movement of 10 SVs in a cell in thezplane was tracked over 100 time steps and then cross-correlated. For comparison, linear-dependent and random trajectories were created and plotted. The bar plot depicts the averaged correlation coefficients across three cells. Data are expressed as mean±s.e.m., ****P<0.0001 (Student’st-test). Figure 1: SVs undergo highly correlated movement that coincides with cortical F-actin translocation towards the plasma membrane following secretagogue stimulation. ( a ) Bovine chromaffin cells expressing NPY-mCherry and lifeact-GFP were examined by TIRF microscopy, imaged at 2 Hz and stimulated with Ba 2+ (2 mM). Fluorescence intensity is depicted in pseudocolour (range: 11,000–28,000 for lifeact-GFP, 2,000–12,000 for NPY-mCherry). Plotted time course of change in NPY-mCherry and lifeact-GFP fluorescence intensity (FI). Scale bar, 5 μm. ( b ) 3D rendering of vesicle trajectories and actin structures over time, highlighting the simultaneous increase in fluorescence intensity for NPY-mCherry and lifeact-GFP. ( c ) Average maximum change in fluorescence intensity (normalized to fluorescence intensity before treatment) for Ba 2+ - or vehicle-treated cells (mean±s.e.m. ; n =10). **** P <0.0001 (Student’s t -test). ( d ) 3D SV trajectories before and at indicated time points during stimulation. Colour code indicates z position. ( e ) Time course of percentage vesicles moving simultaneously towards the plasma membrane. Scoring was based on the percentage of vesicles that moved more than 50 nm in a sliding 10-s interval. ( f ) Multi-cross-correlation analysis of lateral vesicle movement before and at indicated time points during stimulation. Movement of 10 SVs in a cell in the z plane was tracked over 100 time steps and then cross-correlated. For comparison, linear-dependent and random trajectories were created and plotted. The bar plot depicts the averaged correlation coefficients across three cells. Data are expressed as mean±s.e.m., **** P <0.0001 (Student’s t -test). Full size image Highly correlated SV movement towards the plasma membrane We then investigated the three-dimensional (3D) motion of individual NPY-mCherry-labelled SVs in cells before and after stimulation. To obtain z positions, we converted TIR-fluorescence intensities into z coordinates [7] . 3D particle tracking of SVs revealed a significant increase in the number of vesicles undergoing translocation towards the plasma membrane within the first 30 s following stimulation ( Fig. 1d ). The bulk of this translocation was transient, as vesicles that did not undergo fusion returned towards their initial position away from the plasma membrane ( Fig. 1d ). Interestingly, more than 80% of the vesicles present in the TIRF plane moved simultaneously towards the plasma membrane shortly after stimulation ( Fig. 1e ). We performed a multi-cross-correlation analysis of vesicle movement along the vertical axis ( z ) on multiple vesicles ( n =10) and determined correlation coefficients (45 per cell) before and during stimulation. This analysis revealed a high level of cross-correlation 30 s after the onset of stimulation ( Fig. 1f ). This correlation was not detected before or 120 s after stimulation, highlighting the transient nature of this highly synchronized translocation event ( Fig. 1f ). Myosin II inhibition prevents cortical actin and SV translocation We then sought to understand the molecular basis for this coordinated movement of vesicles and cortical actin towards the membrane. As myosin II has previously been implicated in both actin dynamics and neuroexocytosis [23] , we tested whether interfering with its activity and expression levels could block the concerted effect of stimulation on the cortical actin network and vesicle translocation. Preincubation of chromaffin cells with blebbistatin (10 μM for 20 min) completely prevented the joint actin/vesicle movement towards the plasma membrane ( Fig. 2a,b , Supplementary Movie 1 ). Similarly, the short hairpin RNA (shRNA) knockdown of myosin II ( Fig. 2b,c , Supplementary Fig. 3 ) resulted in a complete inhibition of these effects, whereas scrambled RNA-transfected cells exhibited the same displacement as non-shRNA-treated cells ( Fig. 2d ). To assess the direct effect of actin depolymerization on the translocation of SVs and actin towards the plasma membrane, cells were preincubated with cytochalasin-D (2 μM) for 20 min and stimulated. We found that both cortical actin network and SV translocation towards the plasma membrane were reduced in comparison with control cells, but were still significantly greater than in vehicle-treated cells, displaying an intermediary phenotype ( Fig. 2d ). Importantly, single-vesicle 3D analysis confirmed that both blebbistatin and myosin II knockdown interfered with the translocation of cortical actin and SVs to the plasma membrane ( Fig. 2e ), and consequently with the synchronicity of their movement ( Fig. 2f ). Accordingly, the high level of correlation between vesicle movements detected in control cells expressing scrambled RNA was completely lost in response to preincubation with blebbistatin or myosin II knockdown ( Fig. 2g ). Overall, this indicates that myosin II is necessary for the activity-dependent translocation of cortical F-actin and the coordinated movement of SVs towards the plasma membrane. 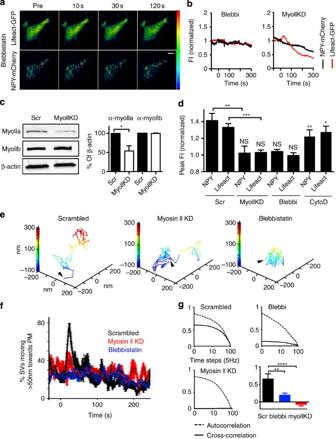Figure 2: Pharmacological inhibition or knockdown of myosin II abolishes concerted movement of SVs and F-actin towards the plasma membrane. (a) Bovine chromaffin cells expressing NPY-mCherry and lifeact-GFP were pretreated for 20 min with blebbistatin (10 μM) and then examined by TIRF microscopy, imaged at 2 Hz and stimulated with Ba2+. Scale bar, 5 μm. (b) Time course of change in fluorescence intensity (FI) for cells treated with blebbistatin and myosin II knockdown as indicated in the figure. (c) Western blot of myosin IIa and myosin IIb following knockdown of myosin IIa in bovine MDBK cells transfected with either scrambled or shRNA-targeting myosin IIa. The level of myosin IIa or IIb is expressed as a percentage of β-actin and normalized to scramble control (mean±s.e.m., 53.49±14.03n=3, and 100.1±0.61n=3; NSP>0.05, *P<0.05). (d) Average maximum change in fluorescence intensity (normalized to fluorescence intensity before treatment) elicited by Ba2+in blebbistatin-treated cells (n=6), cytochalasin-D-treated cells (n=6) myosin II-knockdown cells (n=8) or scrambled RNA-transfected cells (n=8). (mean±s.e.m.) Symbols above bars indicate statistic comparison with vehicle treatment. NSP>0.05, *P<0.05,**P<0.01, ***P<0.001 (Student’st-test). (e) 3D SV trajectories during Ba2+stimulation for myosin II-knockdown cells, cells transfected with scrambled RNA and cells pretreated with blebbistatin. Colour code indicateszposition. (f) Time course of percentage vesicles moving simultaneously towards the plasma membrane. Scoring was based on the percentage of vesicles that moved more than 50 nm in a 10-s interval. (g) Multi-cross-correlation analysis of lateral vesicle movement during stimulation. Movement of 10 vesicles in a cell in thezplane was cross-correlated over 100 time steps (0.2 s). Averaged correlation coefficients for SV trajectories 30 s after the onset of stimulation are depicted in the lower right graph. (mean±s.e.m.,n=3 cells) **P<0.01, ****P<0.0001 (Student’st-test). Figure 2: Pharmacological inhibition or knockdown of myosin II abolishes concerted movement of SVs and F-actin towards the plasma membrane. ( a ) Bovine chromaffin cells expressing NPY-mCherry and lifeact-GFP were pretreated for 20 min with blebbistatin (10 μM) and then examined by TIRF microscopy, imaged at 2 Hz and stimulated with Ba 2+ . Scale bar, 5 μm. ( b ) Time course of change in fluorescence intensity (FI) for cells treated with blebbistatin and myosin II knockdown as indicated in the figure. ( c ) Western blot of myosin IIa and myosin IIb following knockdown of myosin IIa in bovine MDBK cells transfected with either scrambled or shRNA-targeting myosin IIa. The level of myosin IIa or IIb is expressed as a percentage of β-actin and normalized to scramble control (mean±s.e.m., 53.49±14.03 n =3, and 100.1±0.61 n =3; NS P >0.05, * P <0.05). ( d ) Average maximum change in fluorescence intensity (normalized to fluorescence intensity before treatment) elicited by Ba 2+ in blebbistatin-treated cells ( n =6), cytochalasin-D-treated cells ( n =6) myosin II-knockdown cells ( n =8) or scrambled RNA-transfected cells ( n =8). (mean±s.e.m.) Symbols above bars indicate statistic comparison with vehicle treatment. NS P >0.05, * P <0.05,** P <0.01, *** P <0.001 (Student’s t -test). ( e ) 3D SV trajectories during Ba 2+ stimulation for myosin II-knockdown cells, cells transfected with scrambled RNA and cells pretreated with blebbistatin. Colour code indicates z position. ( f ) Time course of percentage vesicles moving simultaneously towards the plasma membrane. Scoring was based on the percentage of vesicles that moved more than 50 nm in a 10-s interval. ( g ) Multi-cross-correlation analysis of lateral vesicle movement during stimulation. Movement of 10 vesicles in a cell in the z plane was cross-correlated over 100 time steps (0.2 s). Averaged correlation coefficients for SV trajectories 30 s after the onset of stimulation are depicted in the lower right graph. (mean±s.e.m., n =3 cells) ** P <0.01, **** P <0.0001 (Student’s t -test). Full size image One plausible explanation for these phenomena is that the contractility of cortical F-actin brings the cortical actin network and its associated vesicles into closer proximity with the plasma membrane. Acute blebbistatin treatment translocates cortical actin and SVs To investigate this hypothesis, we examined the effect of acute blebbistatin treatment on the fluorescence intensity of NPY-mCherry and lifeact-GFP in unstimulated cells. We predicted that if myosin II contractility were responsible for bringing cortical actin and the plasma membrane into closer proximity with one another, then the fluorescence intensity would decrease following exposure to blebbistatin. To our surprise, we found that the intensity of both the lifeact-GFP and NPY-mCherry fluorescence increased in response to blebbistatin treatment ( Fig. 3a ) to a degree that was comparable to that associated with Ba 2+ stimulation. Lifeact-GFP fluorescence intensity increased by 24±2.5% ( n =6) and NPY-mCherry fluorescence intensity by 41±9% ( n =6; Fig. 3b and Fig. 1c ). This suggested that relaxation, rather than contractility, might be responsible for bringing the cortical network closer to the plasma membrane. 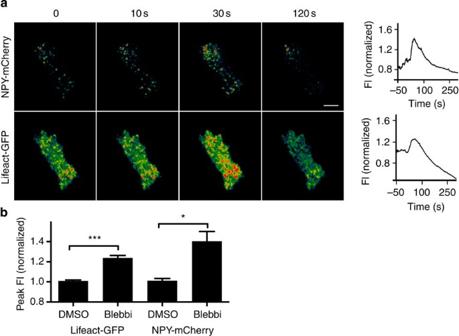Figure 3: Acute myosin II inhibition results in the translocation of F-actin and SVs towards the plasma membrane. (a) Bovine chromaffin cells expressing NPY-mCherry and lifeact-GFP were examined by TIRF microscopy, imaged at 0.5 Hz and treated acutely with blebbistatin (t=0). Fluorescence intensity is depicted in pseudocolour (Range: 12,000–34,000 for lifeact-GFP, 3,800–16,000 for NPY-mCherry). Scale bar, 5 μm. Right panels: time course of change in NPY-mCherry and lifeact-GFP fluorescence intensities (FI) for the cells depicted on the left. (b) Average maximum change in fluorescence intensity for lifeact-GFP and NPY-mCherry after blebbistatin treatment (n=6) or in dimethylsulphoxide (DMSO)-treated controls (mean±s.e.m.,n=4) *P<0.05, ***P<0.001 (Student’st-test). Figure 3: Acute myosin II inhibition results in the translocation of F-actin and SVs towards the plasma membrane. ( a ) Bovine chromaffin cells expressing NPY-mCherry and lifeact-GFP were examined by TIRF microscopy, imaged at 0.5 Hz and treated acutely with blebbistatin ( t =0). Fluorescence intensity is depicted in pseudocolour (Range: 12,000–34,000 for lifeact-GFP, 3,800–16,000 for NPY-mCherry). Scale bar, 5 μm. Right panels: time course of change in NPY-mCherry and lifeact-GFP fluorescence intensities (FI) for the cells depicted on the left. ( b ) Average maximum change in fluorescence intensity for lifeact-GFP and NPY-mCherry after blebbistatin treatment ( n =6) or in dimethylsulphoxide (DMSO)-treated controls (mean±s.e.m., n =4) * P <0.05, *** P <0.001 (Student’s t -test). Full size image Stimulation reduces cortical actin network tension To investigate this, we then sought direct evidence that stimulators of neurotransmitter release induce cortical relaxation. First, we examined the impact on tension at focal adhesions, sites where actomyosin physically associates with integrin adhesion complexes [24] , [25] , [26] . To this end, we expressed a fluorescence resonance energy transfer (FRET)-based vinculin tension sensor (VINTS) [27] , [28] in chromaffin cells. VINTS consists of vinculin head and tail domains with a tension-sensing module inserted between these domains. The tension-sensing module contains monomeric teal fluorescent protein (mTFP) [29] and the yellow fluorescent protein mVenus separated by a molecular spring. This spring stretches in response to molecular tension and its stretch can be measured as a decrease in energy transfer. To measure changes in FRET efficiency, we carried out sensitized emission FRET measurements. The measured FRET index for VINTS-expressing cells was 0.135±0.0064 ( n =7) in comparison with 0.309±0.009 ( n =4) for VINTL, a chimeric construct that lacks the tail domain of vinculin and cannot sense tension, confirming that the sensor is under a degree of tension in resting cells. Stimulation caused a transient increase in sensitized emission FRET in the VINTS construct, consistent with molecular relaxation of the tension sensor; in contrast, VINTL displayed no change in FRET ( Fig. 4a,b ). Consistent with a role for myosin II in generating force, blebbistatin inhibition (FRET index: 0.185±0.023, n =4) or knockdown (FRET index: 0.21±0.017, n =4) of myosin II reduced the tension in resting cells ( Fig. 4c ). Moreover, the stimulation of both myosin II knockdown- and blebbistatin-treated cells did not produce any further reduction in tension ( Fig. 4c ). Thus, pre-existing myosin II activity is necessary for stimulation to cause relaxation across vinculin. This suggests that myosin II inhibition might be key to the physical relaxation of the cell cortex induced by stimulation. 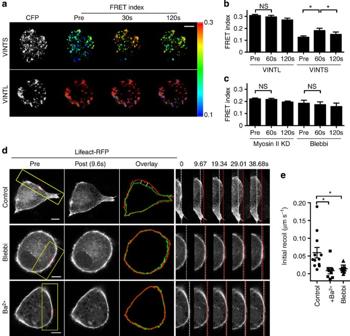Figure 4: Secretagogue stimulation elicits a myosin II-dependent loss in cortical actin network tension. (a) FRET imaging of VINTS and VINTL in chromaffin cells before and during stimulation. Cells expressing VINTS or VINTL were examined by TIRF microscopy. The left panels show mTFP fluorescence before stimulation, and the middle and right panels show the FRET index in pseudo colour at the indicated times before and during stimulation with Ba2+. Scale bar: 5 μm (b) FRET indices of VINTS (n=7) and VINTL (n=4) at indicated times before and during stimulation with Ba2+. (mean±s.e.m., NSP>0.05, *P<0.05, pairedt-test for comparison within VINTS/VINTL, otherwise Student’st-test). (c) FRET indices of VINTS in blebbistatin-treated (n=4) and myosin II-knockdown chromaffin cells (n=4) before and during stimulation with Ba2+. (mean±s.e.m. NSP>0.05, pairedt-test). (d) Laser ablation of control, blebbistatin-treated and Ba2+-stimulated bovine chromaffin cells transfected with lifeact-RFP. Images show the cells before and 10 s after ablation. The overlay represents the position of the cortical actin network before (green) and after (red) ablation Scale bar, 5 μm. The ablation site is indicated by a red square. The image sequences depict the cortical actin network recoil after ablation. The white dashed lines indicate starting positions, and the red dashed lines the expansion after laser ablation. (e) Initial recoil, as measured by the instantaneous rate of cortical actin network relaxation att=0, was reduced in both blebbistatin-treated (n=9) and Ba2+-stimulated cells (n=8) in comparison with controls (n=12). (mean±s.e.m.) *P<0.05 (Student’st-test). Figure 4: Secretagogue stimulation elicits a myosin II-dependent loss in cortical actin network tension. ( a ) FRET imaging of VINTS and VINTL in chromaffin cells before and during stimulation. Cells expressing VINTS or VINTL were examined by TIRF microscopy. The left panels show mTFP fluorescence before stimulation, and the middle and right panels show the FRET index in pseudo colour at the indicated times before and during stimulation with Ba 2+ . Scale bar: 5 μm ( b ) FRET indices of VINTS ( n =7) and VINTL ( n =4) at indicated times before and during stimulation with Ba 2+ . (mean±s.e.m., NS P >0.05, * P <0.05, paired t -test for comparison within VINTS/VINTL, otherwise Student’s t -test). ( c ) FRET indices of VINTS in blebbistatin-treated ( n =4) and myosin II-knockdown chromaffin cells ( n =4) before and during stimulation with Ba 2+ . (mean±s.e.m. NS P >0.05, paired t -test). ( d ) Laser ablation of control, blebbistatin-treated and Ba 2+ -stimulated bovine chromaffin cells transfected with lifeact-RFP. Images show the cells before and 10 s after ablation. The overlay represents the position of the cortical actin network before (green) and after (red) ablation Scale bar, 5 μm. The ablation site is indicated by a red square. The image sequences depict the cortical actin network recoil after ablation. The white dashed lines indicate starting positions, and the red dashed lines the expansion after laser ablation. ( e ) Initial recoil, as measured by the instantaneous rate of cortical actin network relaxation at t =0, was reduced in both blebbistatin-treated ( n =9) and Ba 2+ -stimulated cells ( n =8) in comparison with controls ( n =12). (mean±s.e.m.) * P <0.05 (Student’s t -test). Full size image To validate our results, we used frequency-domain fluorescence lifetime imaging. The donor only control (mTFP) yielded a lifetime of 2.5 ns, in agreement with previous reports [29] . VINTL produced a lifetime of 2±0.04 ns ( n =4), which corresponds to a FRET efficiency of 22.5% (ref. 27 ). An average lifetime of 2.25±0.06 ns ( n =4), equivalent to 9.5% FRET efficiency, was obtained for VINTS ( Supplementary Fig. 2a,c ). Ba 2+ stimulation elicited a significant reduction in VINTS lifetime but not in the lifetime of the VINTL control ( Supplementary Fig. 2b,c ). As physical tension through the cell substrate adhesion sites was reduced on stimulation, we next sought to investigate whether cortical tension was affected globally by stimulation, beyond the specific context of focal adhesions. To measure cortical tension, we used laser nanoablation [19] to cut the cortical actin network. We then measured the instantaneous rate of recoil as an index of cortical actin network tension [30] . These laser nanoablation experiments were performed on cells that were untreated (control), preincubated with blebbistatin or stimulated with Ba 2+ . Control cells displayed significant instantaneous recoil (speed of recoil immediately after ablation) of the cortical actin network (0.06±0.015 μm s −1 , n =12) after it was severed by the laser nanoscissors ( Fig. 4d,e , Supplementary Movie 3 ), consistent with the presence of basal cortical tension. In contrast, the instantaneous rate of recoil (indicating tension) was reduced in cells that were pretreated with blebbistatin (0.014±0.0036 μm s −1 , n =9) or stimulated with Ba 2+ (0.009±0.0009 μm s −1 , n =8; Fig. 4d,e , Supplementary Movies 4 and 5 ). Blebbistatin reduces the number of early fusion events We next tested whether myosin II inhibition had an effect on the rate of neurosecretory vesicle fusion during the early phase of stimulation, coincident with the simultaneous approach of the cortical actin and SVs to the plasma membrane. To this end, we analysed NPY-emerald(em)GFP-positive vesicle fusions in stimulated cells that were either untreated, blebbistatin-treated or co-transfected with either myosin II-shRNA or scrambled RNA. Fusion events were counted within the first 30 s of stimulation. Fusion events were detected as an increase in fluorescence intensity in TIR-illumination followed by the disappearance of a vesicle [31] , [32] ( Fig. 5a ). The number of fusions per cell membrane area was significantly reduced during this period in both blebbistatin-treated and myosin II-knock-down cells in comparison with untreated or scrambled RNA-transfected cells ( Fig. 5b ). Similarly, using amperometry, we observed a significant drop in the number of exocytic events for cells treated with blebbistatin (36±5.6 spikes, n =6 cells) in comparison with control cells (100.7±15.8 spikes, n =10 cells; Fig. 5c ). Interfering with myosin II function therefore reduces the number of exocytic events elicited in the early phase of secretagogue stimulation. 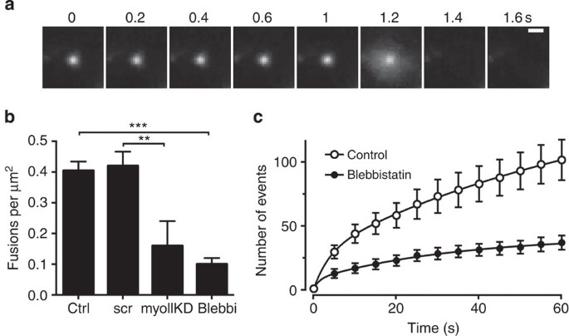Figure 5: The number of secretory fusions at the onset of stimulation is reduced in myosin II-inhibited cells. (a) Effect of myosin II inhibition on the number of vesicle fusions within the first 30 s of stimulation in bovine chromaffin cells. Cells were imaged in TIRF at 5 Hz and stimulated with Ba2+. Fusions were scored by the disappearance of a vesicle accompanied by a flash in fluorescence intensity. Scale bar, 1 μm. (b) Counts of vesicle fusions in untreated, scrambled RNA-, myosin II knockdown- and blebbistatin-treated cells. Data are means±s.e.m. **P<0.01, ***P<0.001, (Student’st-test). (c) Time course of release events per 5-s interval measured using amperometry in blebbistatin-treated and control cells following stimulation. Figure 5: The number of secretory fusions at the onset of stimulation is reduced in myosin II-inhibited cells. ( a ) Effect of myosin II inhibition on the number of vesicle fusions within the first 30 s of stimulation in bovine chromaffin cells. Cells were imaged in TIRF at 5 Hz and stimulated with Ba 2+ . Fusions were scored by the disappearance of a vesicle accompanied by a flash in fluorescence intensity. Scale bar, 1 μm. ( b ) Counts of vesicle fusions in untreated, scrambled RNA-, myosin II knockdown- and blebbistatin-treated cells. Data are means±s.e.m. ** P <0.01, *** P <0.001, (Student’s t -test). ( c ) Time course of release events per 5-s interval measured using amperometry in blebbistatin-treated and control cells following stimulation. Full size image Myosin II acts upstream of Munc18-1-dependent docking To examine whether the reduction in fusion events resulted from reduced SV docking in response to stimulation, we used PC12 cells engineered to knock down Munc18-1 and Munc18-2 (DKD-PC12 cells) [31] , which have been shown to exhibit defective vesicle docking [31] , [33] . Electron microscopy analysis revealed that the number of predocked granules in these cells was significantly reduced in comparison with that in DKD-PC12 cells in which wild-type Munc18-1 (Munc18-1) expression was rescued ( Fig. 6a,b ). However, in both NPY-mCherry-expressing DKD-PC12 cells and Munc18-1 rescued DKD-PC12 cells, barium stimulation resulted in an increase in fluorescence intensity similar to the effect observed in chromaffin cells, indicating SV translocation towards the plasma membrane ( Fig. 6c ). This suggests that Munc18-1 does not control the translocation mechanism that allows both the cortical actin network and tethered SVs to move towards the plasma membrane. We then performed SV tracking before and during stimulation in both PC12-DKD cells and Munc18-1-rescued PC12-DKD cells ( Fig. 6d ) and measured the mean squared displacements (MSDs) of all trajectories to calculate cage radii and to assess vesicle mobility [10] . In the Munc18-1-rescued cells, we found a cage radius of 0.14±0.02 μm ( n =6; Fig. 6e ). On barium stimulation, lateral SV mobility became restricted with a cage radius of 0.07±0.006 μm ( Fig. 6e ), a process that has previously been associated with vesicles docking at the plasma membrane [34] , [35] . However, in control PC12-DKD cells, the SV mobility (cage radius: 0.1714±0.027 μm, n =7, Fig. 6e ) did not change significantly after stimulation (cage radius: 0.1888±0.022 μm), confirming that while SVs were able to translocate towards the plasma membrane they could not undergo docking in the absence of Munc18-1. We then tested whether blebbistatin inhibition could affect SV docking in chromaffin cells and analysed SV movement before and during stimulation ( Fig. 6f ). In control chromaffin cells, we observed a reduction in SV cage size (cage radius: 0.267±0.021 μm, n =6) on stimulation (cage radius: 0.204±0.011 μm, Fig. 6f,g ) indicative of successful docking. However, in cells pretreated with blebbistatin, SV mobility (cage radius: 0.2195±0.025 μm, n =4) was not affected by stimulation (cage radius 0.268±0.028 μm; Fig. 6f,g ), suggesting that none of the vesicles could undergo docking. These data suggest that relaxation-driven translocation of SVs towards the plasma membrane is a pre-requisite for their activity-dependent docking. 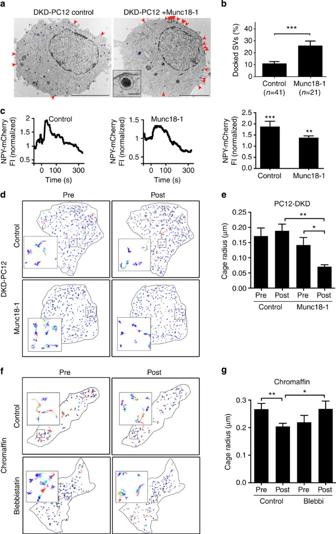Figure 6: Munc18-1 controls SV docking but not myosin II-dependent SV translocation to the plasma membrane. (a) DKD-PC12 cells were transfected with Munc18-1-emGFP or emGFP, fixed and processed for electron microscopy. The insert shows a docked SV. (b) DKD-PC12 control cells were found to contain a significantly reduced fraction of docked SVs relative to Munc18-1-emGFP-expressing cells (10.92±1.73,n=41 and 25.9±4.061,n=21, mean±s.e.m. ***P<0.001, Student’st-test). (c) DKD-PC12 cells expressing NPY-mCherry were examined by TIRF microscopy, imaged at 2 Hz and stimulated with Ba2+(2 mM). Plotted time course of change in NPY-mCherry fluorescence intensity (FI). NPY-mCherry-FI increases in both Munc18-1-rescued and control DKD-PC12 (1.38±0.08,n=6 and 1.708± 0.24,n=4, mean±s.e.m.) **P<0.01, ***P<0.001, (Student’st-test) cells following stimulation with Ba2+, indicating the transition of SV towards the plasma membrane. (d,e) Tracking of SVs in DKD-PC12 cells expressing NPY-mCherry. Cells were imaged by TIRF microscopy at 10 Hz. NPY-mCherry-positive SVs were tracked, and their MSD and cage size analysed. Track MSD is displayed as a colour code. Following stimulation the MSD of SVs and the average cage radius become restricted (0.14±0.02 μm,n=6 and 0.07±0.025 μm,n=6, mean±s.e.m.), *P<0.05, **P<0.01, (Student’st-test) in Munc18-1-rescued DKD-PC12 cells, indicating SV docking. In control DKD-PC12 cells, mobility is not reduced on stimulation (cage radius before stimulation: 0.17±0.027 μm,n=7, cage radius after stimulation: 0.189±0.022 μm,n=7, mean±s.e.m.), *P<0.05, **P<0.01 (Student’st-test), indicating the absence of functional docking. (f,g) Tracking of SVs in chromaffin cells expressing NPY-mCherry. Cells were imaged by TIRF microscopy at 10 Hz. NPY-mCherry-positive SVs were tracked, and their MSD and cage size analysed. The MSD and cage size of SVs in control chromaffin cells becomes restricted on stimulation (prestimulation: 0.267±0.021 μm,n=6, post stimulation: 0.2044±0.012 μm,n=6, mean±s.e.m.), *P<0.05, **P<0.01, (Student’st-test), indicating docking at the plasma membrane. The MSD and cage radius of SVs in cells pretreated with blebbistatin does not change significantly in comparison with control cells on stimulation (cage radius before 0.22±0.025 μm,n=4, cage radius after: 0.268±0.029 μm,n=4, mean±s.e.m.). Figure 6: Munc18-1 controls SV docking but not myosin II-dependent SV translocation to the plasma membrane. ( a ) DKD-PC12 cells were transfected with Munc18-1-emGFP or emGFP, fixed and processed for electron microscopy. The insert shows a docked SV. ( b ) DKD-PC12 control cells were found to contain a significantly reduced fraction of docked SVs relative to Munc18-1-emGFP-expressing cells (10.92±1.73, n =41 and 25.9±4.061, n =21, mean±s.e.m. *** P <0.001, Student’s t -test). ( c ) DKD-PC12 cells expressing NPY-mCherry were examined by TIRF microscopy, imaged at 2 Hz and stimulated with Ba 2+ (2 mM). Plotted time course of change in NPY-mCherry fluorescence intensity (FI). NPY-mCherry-FI increases in both Munc18-1-rescued and control DKD-PC12 (1.38±0.08, n =6 and 1.708± 0.24, n =4, mean±s.e.m.) ** P <0.01, *** P <0.001, (Student’s t -test) cells following stimulation with Ba 2+ , indicating the transition of SV towards the plasma membrane. ( d , e ) Tracking of SVs in DKD-PC12 cells expressing NPY-mCherry. Cells were imaged by TIRF microscopy at 10 Hz. NPY-mCherry-positive SVs were tracked, and their MSD and cage size analysed. Track MSD is displayed as a colour code. Following stimulation the MSD of SVs and the average cage radius become restricted (0.14±0.02 μm, n =6 and 0.07±0.025 μm, n =6, mean±s.e.m. ), * P <0.05, ** P <0.01, (Student’s t -test) in Munc18-1-rescued DKD-PC12 cells, indicating SV docking. In control DKD-PC12 cells, mobility is not reduced on stimulation (cage radius before stimulation: 0.17±0.027 μm, n =7, cage radius after stimulation: 0.189±0.022 μm, n =7, mean±s.e.m. ), * P <0.05, ** P <0.01 (Student’s t -test), indicating the absence of functional docking. ( f , g ) Tracking of SVs in chromaffin cells expressing NPY-mCherry. Cells were imaged by TIRF microscopy at 10 Hz. NPY-mCherry-positive SVs were tracked, and their MSD and cage size analysed. The MSD and cage size of SVs in control chromaffin cells becomes restricted on stimulation (prestimulation: 0.267±0.021 μm, n =6, post stimulation: 0.2044±0.012 μm, n =6, mean±s.e.m. ), * P <0.05, ** P <0.01, (Student’s t -test), indicating docking at the plasma membrane. The MSD and cage radius of SVs in cells pretreated with blebbistatin does not change significantly in comparison with control cells on stimulation (cage radius before 0.22±0.025 μm, n =4, cage radius after: 0.268±0.029 μm, n =4, mean±s.e.m.). Full size image In this study, we investigated the mechanism controlling the activity dependent translocation of SVs to the plasma membrane. We discovered that myosin II maintains the cortical actin network in tension at rest and that secretagogue stimulation elicits a relaxation that drives the cortical actin network and tethered SVs towards the plasma membrane. We further show that following this recruitment to the plasma membrane SVs undergo Munc18-1-dependent docking and subsequent fusion. Before stimulation, only a small number of SVs are primed and ready for an initial burst of fusion events [3] , [4] , [5] . Most SVs in the vicinity of the plasma membrane are tethered to the cortical actin network [36] and the displacement of the latter towards the plasma membrane provides an efficient way to bring SVs to their docking sites. Both partial actin depolymerization immediately after stimulation [37] as well as N-WASP- and Cdc42-dependent actin polymerization [7] , [38] have been shown to contribute to neuroexocytosis, demonstrating the pleiotropic role of the cortical actin network as both a retaining barrier and a means of SV transport. Myosin II has previously been implicated in a number of steps leading to SV fusion, with most studies showing that it is directly involved in controlling fusion pore dynamics [12] , [14] , [17] , [39] . Our data add another layer to our understanding of the function of myosin II in exocytosis. By maintaining tension of the cortical actin network [18] , [19] , [40] in unstimulated cells, myosin II retains most SVs away from the plasma membrane. This is in good agreement with previous reports showing that the cortical actin network acts as a barrier, preventing the majority of vesicles from accessing the plasma membrane in resting conditions [2] , [9] . To the best of our knowledge, our study is the first to demonstrate that relaxation of the cortical actin network is the main driving force that allows SVs to be translocated and recruited to the plasma membrane. This has been demonstrated using two independent methods including nanoscissors [19] and direct measurement of the tension applied to the FRET tension sensor VINTS [27] . Our results suggest that the myosin II-maintained cortical actin network tension produces a dynamic equilibrium of forces measurable at the level of focal adhesion sites. On secretagogue stimulation, actomyosin II relaxation results in a force that provides elastic displacement, allowing SVs to move towards the plasma membrane. The molecular mechanism causing such relaxation is likely to involve inhibition of myosin II, as acute blebbistatin treatment is able to mimic the effect of stimulation in causing cortical actin network relaxation and promoting a transient movement of SVs towards the plasma membrane. Furthermore, longer pretreatment with blebbistatin or myosin II knockdown prevented secretatogue-induced translocations of cortical actin network and associated SVs. The molecular mechanism underpinning this stimulation-induced acute inhibition of myosin II function is currently unknown but Ca 2+ (ref. 41 ) and Rho-kinases such as ROCK I and II (ref. 42 ) are likely regulating candidates. However, more work is needed to address this issue. Another unknown is how such a casting net mechanism can lead SVs to pre-existing release sites on the plasma membrane. Recent evidence suggests that SVs can organize their own release sites on reaching the plasma membrane [32] , [43] . Indeed, syntaxin-1 molecules have been shown to concentrate under docked vesicles before fusion, suggesting that a pool of plasma membrane syntaxin-1 can be recruited by an unknown mechanism under SVs [43] . Another possible contributing factor could involve translocated actin exerting an effect on the domain organization of the plasma membrane [44] leading to efficient docking as previously speculated [45] . Consistent with earlier key reports using TIRF microscopy, we also found that both chromaffin cell and PC12 cell SVs become restricted in their lateral movement following stimulation, indicating that they are undergoing docking [34] , [35] . Importantly, we could not observe such a restriction in movement in DKD-PC12 cells. However, SVs did translocate to the plasma membrane in response to stimulation, demonstrating that (1) Munc18-dependent docking [46] occurs downstream of SVs and (2) activity-dependent translocation of the cortical actin network and tethered SVs does not require Munc18-1. The fact that blebbistatin inhibits both the translocation of SVs towards the plasma membrane and the restriction of the vesicles undergoing docking further confirms that such translocation is upstream of docking. It is worth noting that even though blebbistatin blocks the initial burst of catecholamine release events, a slower wave of release is unaffected by myosin II inhibition. This is probably due to other cytoskeletal effects, as described previously [9] . It is also important to note that myosin II is involved in regulating fusion pore dynamics, which also affects the release process [12] , [17] , [47] . In conclusion, our results reveal that myosin II plays a pivotal role in maintaining cortical actin network tension, and that secretagogue stimulation promotes the relaxation of this network, driving the coordinated movement of actin-tethered SVs towards the plasma membrane. On reaching the plasma membrane, Munc18-1 coordinates the docking process before fusion. This novel function of the cortical actomyosin II network allows for the synchronized translocation of the majority of SVs visible in the TIRF plane towards the plasma membrane, thereby maximizing the efficiency of neurotransmitter and hormone release in response to stimulation. Cell culture and reagents Chromaffin cells were isolated from bovine adrenal glands [48] , [49] and maintained in Dulbecco's modified Eagle’s medium supplemented with 10% serum supreme, 2.5 μg ml −1 fungizone, 50 μg ml −1 gentamycin and 10 mM HEPES on 0.1 mg ml −1 poly- D -lysine-coated culture dishes (MatTek Corporation). Cells were transfected using electroporation (Amaxa Basic Nucleofector Kit for primary neurons (Lonza), Program X-001) and cultured at 37 °C/5% CO 2 for at least 24 h before experimentation. Transfected cells were plated onto poly- D -lysine-coated glass-bottomed culture dishes (MatTek Corporation) and processed for imaging 48–72 h post transfection. Lifeact-GFP [50] was provided by Roland Wedlich Soldner (MPI Biochemistry, Martinsried), GPI-anchored GFP (GFP–GPI) was a gift from Kai Simons (MPI-CBG, Dresden). pCMV-neuropeptide Y-mCherry (NPY-mCherry) was generated from pCMV-NPY-emerald GFP provided by Shuzo Sugita (University of Toronto). In brief, mCherry was amplified from pmCherry-C1 (Takara Bio Inc.) by PCR using the following primers: forward, 5′- ATCGATAAGCTCATGGTGGCAAGGGCGAG -3′; and reverse, 5′- CAAGTAAAACCTCTACAAATGTGGTATGGC -3′. It was then subcloned into pCMV-NPY-emerald GFP using ClaI and BamHI, replacing emerald GFP [10] . Myosin II knockdown Verification of myosin IIa knockdown was performed using the bovine MDBK cell line (Sigma). Cells were tranfected by lipofectaime LTX (Life Technologies) with scrambled and myosin IIa targeting shRNA 5′- AGAAGGTGAAGGTGAACAAGGATGATATC -3′ (Origene, Myh9 NM_001192762.1). Twenty-four hours post transfection, the cells were grown in medium containing 1 μg ml −1 of Puromycin for selection. Cells were processed and knockdown efficiency was determined using SDS-polyacrylamide gel electrophoresis and western blotting 72 h post transfection. Myosin IIa or myosin IIb was detected using a polyclonal antibody (Sigma-Aldrich) and β-actin (Abcam) was used as a loading control. Analysis of knockdown efficiency was determined using Image J. TIRF microscopy Transfected cells on glass-bottomed culture dishes (MatTek) were visualized with a TIRF microscope (Marianas, SDC EverestTM, Intelligent Imaging Innovations Inc.) fitted with a × 100 oil immersion objective (NA=1.46, Carl Zeiss Pty) using EMCCD cameras (QuantEM 512sc) and Slidebook software (version 5.5). Cells were bathed in Buffer A, before the addition of 2 mM BaCl 2 or 100 μM nicotine+2 mM CaCl 2 . Time-lapse movies were captured for the indicated period and frequency. When cytoskeletal inhibitors were used, these were preincubated with the cells for 20 min before imaging. Frequency-domain FLIM images were obtained on the same microscope using a Princeton instruments PI-MAX4:1024 ICCD camera and images were calculated using Slidebook 5.5 (3i). Single-vesicle trajectories Individual SV trajectories were obtained using the manual tracking function of the Slidebook software (version 5.5). For z shift analysis, trajectories were obtained using Imaris (Version 7.3.1, Bitplane AG) spot and tracking features. Particle tracking of NPY-mCherry-labelled SVs was performed on previously acquired TIRF images utilizing the spot-tracking function of Imaris. SVs were tracked for 3 min following Ba 2+ stimulation. The spot diameter was 0.30 μm and the vesicles were selected based on local contrast thresholding after background subtraction. Tracking was performed using the built-in autoregressive motion model with maximum displacement of 0.5 μm per time step and a gap size of 1 frame. z positions were calculated as described previously [7] . MSD was calculated for each vesicle over incrementing time intervals and then averaged [34] . To characterize SG mobility, MSD data were fitted to various diffusion models; best fits were obtained when a confined diffusion model was assumed [51] . In this model, the MSD is described as follows and provides a second-order approximation of vesicle diffusion within a finite space or cage: A 1 and A 2 are constants determined by the cage geometry with A 1 =0.99 and A 2 =0.85 for circular cages [51] , [52] . D is the diffusion coefficient of a particle within the cage and r is the radius of the circular cage in which an infinitesimally small particle is free to diffuse with diffusion coefficient D α . Only SVs tracked for >40 consecutive frames were considered. Cross-correlation analysis Bovine chromaffin cells were imaged at 5 Hz and NPY-mEmerald labelled SVs were tracked manually using Slidebook 5.5 (Intelligent Imaging Innovations) before and during stimulation. The track length was 100 frames and at least 10 vesicles were tracked per cell. Intensity profiles of individual vesicles were used to obtain z positions for each time point resulting in z trajectories for each vesicle. Multi-cross-correlation analysis was performed using Matlab’s xcorr function. The cross-correlation values for each analysis were averaged and plotted. FRET metrics and normalizations FLIM measurements are reported as FRET efficiency: with τ DA being the donor (mTFP) lifetime in presence of the acceptor (mVenus) and τ D being the donor lifetime without acceptor. For sensitized emission FRET measurements, we first calculated the spectral bleedthrough for mTFP. For FRET measurements, we acquired images in the mTFP and FRET channel and performed background subtraction and channel alignment before FRET analysis. The FRET index was calculated using the following equation [53] : where I FRET and I mTFP correspond to the background subtracted images of cells expressing VINTS or VINTL. a is the bleedthrough correction coefficient that was obtained by measuring mTFP emission in the mVenus channel. Laser nanoablation Laser nanoablation experiments were performed on a LSM 510 meta Zeiss confocal microscope equipped with a heating stage set to 37 °C for the duration of the time-lapse. Images (300 × 300 pixels, 0.19 μm per pixel) were acquired using a × 63 objective, 1.4 NA oil Plan Apochromat immersion lens at 3 digital magnification and pinhole adjusted to 3 Airy units to obtain optical section 2 μm thick. Time-lapse images were acquired before (two frames) and after (18 frames) ablation with an interval of 10 s per frame. For ablation, a tuneable Ti:Sapphire laser (Chameleon Ultra, Coherent Scientific) tuned to 790 nm was used to ablate cortical actin labelled with lifeact-RFP (red fluorescent protein). A constant circular region of interest, 1.54 μm diameter was marked for each experiment and ablated with 30 iterations of the 790 nm laser with 38% transmission. GFP fluorescence was determined before and after the induced ablation using a 488 nm laser for excitation and a 500–550 nm emission filter, and RFP fluorescence was determined using 543 nm laser excitation and 560 long-pass emission. Image analysis was performed using Imaris. The distance ( d ) between the cortical actin network at the site of ablation before and after ablation was measure as a function of time ( t ). After plotting, the resulting values were fitted to the following equation: The instantaneous recoil (rate of recoil at t =0 s) was then determined as: Instantaneous recoil : The average instantaneous recoil was determined for 8 to 12 cells. Fusion event analysis The fusion of NPY-mCherry/NPY-emGFP-positive SVs with the plasma membrane of the footprint was scored by the disappearance of a labelled SV and a transient local increase in fluorescence intensity following NPY-mCherry/NPY-emGFP release. Amperometry Catecholamine release from single-chromaffin cells was measured using amperometry50 by applying +800 mV to a carbon-fibre electrode (ProCFE, Dagan Corporation), and recording the resultant current (EPC-9 amplifier and Pulse software, HEKA Electronic), sampled at 10 kHz and low-pass filtered at 1 kHz. Spikes were analysed (Mini Analysis, 6.0.1, Synaptosoft) for a period of 60 s. The bath solution contained 140 mM NaCl, 5 mM KCl, 2 mM CaCl 2 , 1 mM MgCl 2 , 5 mM D -glucose and 10 mM HEPES, pH 7.4. The stimulating solution contained 70 mM K + replacing an equimolar amount of NaCl. Experiments were conducted at 35–37 °C using an in-line solution heater (Warner Instruments). Amperometric spikes were selected if spike amplitude exceeded 10 pA. Cells with 10–200 events were used for the analysis. Electron microscopy DKD-PC12 cells expressing Munc18-1-emGFP were seeded on gridded poly- D -lysine-coated glass-bottomed culture dishes (MatTek Corporation). After 24 h, cells were fixed in 2.5% glutaraldehyde in PBS. Sections (50 nm) were cut using an ultramicrotome (UC64; Leica) and imaged using a transmission electron microscope (model 1011; JEOL) equipped with a cooled charge-coupled device camera (Morada; Olympus). All images were processed using Photoshop CS5.1 (Adobe), and figures were compiled with Illustrator CS5.1 (Adobe). How to cite this article: Papadopulos, A. et al . Activity-driven relaxation of the cortical actomyosin II network synchronizes Munc18-1-dependent neurosecretory vesicle docking. Nat. Commun. 6:6297 doi: 10.1038/ncomms7297 (2015).